Mechanism of carrier accumulation in perovskite thin-absorber solar cells Photovoltaic conversion requires two successive steps: accumulation of a photogenerated charge and charge separation. Determination of how and where charge accumulation is attained and how this accumulation can be identified is mandatory for understanding the performance of a photovoltaic device and for its further optimization. Here we analyse the mechanism of carrier accumulation in lead halide perovskite, CH 3 NH 3 PbI 3 , thin-absorber solar cells by means of impedance spectroscopy. A fingerprint of the charge accumulation in high density of states of the perovskite absorber material has been observed at the capacitance of the samples. This is, as far as we know, the first observation of charge accumulation in light-absorbing material for nanostructured solar cells, indicating that it constitutes a new kind of photovoltaic device, differentiated from sensitized solar cells, which will require its own methods of study, characterization and optimization. Nanostructured (NS) solar cells constitute a powerful alternative for the development of the third generation of photovoltaic devices. The second generation, thin-film solar cells, allows in many cases a reduction in production cost in comparison with the first generation, Si solar cells. In the third generation, in addition, an increase in efficiency is potentially attainable [1] . To reduce the cost of photovoltaic devices, an efficient strategy is to relax the quality requirements of the materials forming the device. However, in conventional Si solar cells, high crystal quality is required, as both photogenerated electrons and holes are transported along the same material, and defects act as recombination centres reducing the cell performance. The material quality can be relaxed if just one carrier is transported along one specific material. This is the working principle of sensitized solar cells (SSCs), in which light absorption and carrier transport are decoupled [2] . In SSCs, charge is photogenerated in dye (DSSCs), thin semiconductor (SSSCs) or in a semiconductor quantum dot (QDSSCs), for small semiconductor nanocrystal sensitizers in which the regime of quantum confinement is reached [3] , [4] . The photogenerated charge is quickly injected into two different transport media: one for electrons transport media (ETM), generally a wide band gap semiconductor such as TiO 2 , and the other one for holes (HTM). As only a single carrier is present in the transporting media, the carrier recombination is reduced and less demanding materials can be employed. In this context, the necessity of NS devices arises from the fact that a single-molecular layer or a semiconductor, extremely thin absorber (~nm), cannot completely harvest the incident sunlight. By nanostructuring the electrode, the effective area to be covered by the sensitizer can be increased by several orders of magnitude. In fact, the appearance of these electrodes enormously increased the efficiency of DSSCs [2] . In this sense, the role of NS metal oxide electrodes is well defined in the form of selective electron contact and ETM with high effective surface area to enhance cell harvesting. Since the seminal paper on DSSCs by O'Regan and Grätzel in the early 1990s [2] , the recent demonstration of all-solid NS solar cells with efficiency higher than 10% constitutes one of the most important breakthroughs in this field [5] , [6] , [7] , [8] . Open circuit voltages as high as 1.3 V (ref. 9 ) and efficiencies of 12.3% (refs 7 , 8 ), even higher than that of the record liquid DSSC, have been very recently demonstrated. In this kind of cell, nanoparticles or a thin film of CH 3 NH 3 PbX 3 , with a perovskite crystalline structure (where X is a halogen element I, Cl, Br or a combination), are deposited on a NS semiconductor with or without hole-transporting material (HTM). Lead halide perovskites have already shown great potential in quantum dot-sensitized solar cells with a liquid HTM [10] , [11] . However, it was the recent report on all-solid devices, with easier perspectives for industrialization, that has revolutionized the field of NS photovoltaic devices. However, the working principles of these devices are not completely understood, as there is clear evidence that these devices do not work as the conventional sensitized solar cell, in which both ETM and HTM are needed. Solar cells with lead halide perovskite and no ETM have been prepared with efficiency η =10.9% using Al 2 O 3 NS electrodes in which perovskite cannot photoinject because of a type I band alignment [6] , whereas devices with no HTM and η =5.5% have been prepared by directly contacting the perovskite with an Au contact [12] . In this work, to unveil the working principles of these devices and concretely understand the mechanism of charge accumulation needed for the photovoltaic conversion, a systematic study based on impedance spectroscopy (IS) characterization has been carried out under both dark and illuminated conditions. The direct signature of perovskite light-absorbing material has been observed in the capacitance of the device, indicating charge accumulation in the electronic states of perovskite. In the DSSC, the charge accumulation in the light-absorbing material (the dye) has not been detected by electrochemical measurement, and for QDSSCs it was detected indirectly as a change in the capacitance slope [13] . Here we present the first report of charge accumulation in light-absorbing material for NS solar cells, which is attributed to a density of states (DOS) that is larger in the perovskite absorber than in either ETM or HTM. This fact makes lead halide perovskite solar cells a new type of photovoltaic device halfway between NS and thin-film solar cells. Performance of flat and NS solar cells In order to have a general view of the performance of photovoltaic devices using perovskite as light-absorbing material, different cells with flat and NS electrodes have been prepared using CH 3 NH 3 PbI 3 as the light-absorbing material. CH 3 NH 3 PbI 3 was prepared following the previously reported methods [5] . Briefly, glass covered with a thin film of transparent conductive SnO 2 :F (FTO) was used as the substrate for electrode preparation. A compact layer of TiO 2 was deposited on top of FTO. Electrodes prepared in this way are hereafter called ‘Flat’ electrodes. Two types of NS electrodes were prepared with an additional layer formed by TiO 2 or ZrO 2 nanoparticles. Finally, on these electrodes are sequentially deposited CH 3 NH 3 PbI 3 , spiro-MeOTAD as HTM and Au contact. Details of SEM, TEM and energy-dispersive X-ray spectroscopy (EDXS) characterization of Flat and NS devices can be found in Supplementary Figs S1–S4 . Blank cells prepared exactly in the same way but without perovskite were also prepared. See Methods section for more details on sample preparation. 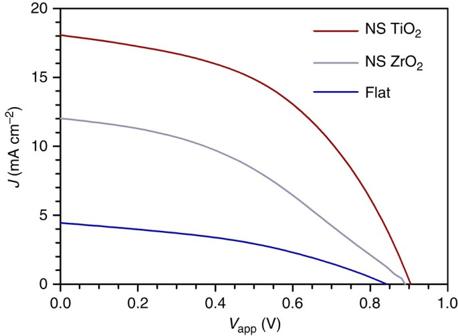Figure 1: Solar cell performance. Current–potentialJ–Vcurves of lead iodine PS with three different electrodes: FTO/compact TiO2(Flat), FTO/compact TiO2/nanostructured TiO2(NS TiO2) and FTO/compact TiO2/nanostructured ZrO2(NS ZrO2). Solar cell parameters and conversion efficiency are summarized inTable 1. Figure 1 shows the current–potential ( J–V ) curves of samples prepared with different electrodes at one-sun illumination. The solar cell parameters, components and geometrical issues of these samples are reported in Table 1 . All the prepared devices exhibit high open circuit potential, V OC . The photocurrent ( J SC ) obtained decreases from NS TiO 2 to NS ZrO 2 to Flat electrode. The light absorption measured for NS ZrO 2 with perovskite electrodes is lower than that for NS TiO 2 electrodes of the same thickness, see Supplementary Fig. S5 . Cells prepared with NS TiO 2 also exhibit higher FF and consequently the highest conversion efficiency of the set, a significant η =7.8%. Samples prepared on the NS ZrO 2 electrode present an appreciable efficiency of 4.2%. It is also interesting that non-negligible efficiency and photocurrent is obtained even for Flat devices, as it has been already seen for other inorganic semiconductors [14] , but not for dyes [15] , because of the high perovskite extinction coefficient. In Supplementary Fig. S6 the results obtained in this work for NS and flat samples are compared with our previous report on all-solid QDSSCs of TiO 2 /Sb 2 S 3 /P3HT (ref. 14 ) to highlight the consistency between them. Figure 1: Solar cell performance. Current–potential J–V curves of lead iodine PS with three different electrodes: FTO/compact TiO 2 (Flat), FTO/compact TiO 2 /nanostructured TiO 2 (NS TiO 2 ) and FTO/compact TiO 2 /nanostructured ZrO 2 (NS ZrO 2 ). Solar cell parameters and conversion efficiency are summarized in Table 1 . Full size image Table 1 Solar cell parameters. Full size table The conduction band of CH 3 NH 3 PbI 3 is situated at −3.93 eV compared with vacuum, whereas TiO 2 is situated around −4 eV, as determined by ultraviolet photoelectron spectroscopy [5] . Therefore, the photogenerated charge in CH 3 NH 3 PbI 3 perovskites can potentially be injected into TiO 2 , as there exists an adequate band alignment. This is not the case for ZrO 2 with a conduction band 0.82 eV higher than the conduction band of TiO 2 (ref. 16 ). ZrO 2 is commonly used as control measurement for the characterization of sensitizers, as no injection into ZrO 2 is observed, in contrast with TiO 2 (ref. 17 ). In fact, no photovoltaic performance was observed for samples prepared with a compact ZrO 2 layer instead of compact TiO 2 , as we have verified experimentally. The electrical differences between TiO 2 and ZrO 2 electrodes have been investigated by three-electrode electrochemical measurements using a liquid electrolyte. Liquid electrolytes are excellent contacts for NS samples, as liquid wets the entire NS surface. Moreover, through the utilization of a redox couple, the Fermi level at the solution can be fixed, and the observed voltage drop is at the semiconductor electrode side. Fig. 2 shows the capacitance of different electrodes formed with a compact layer and a nanoporous layer of TiO 2 and ZrO 2 . It can be observed that the capacitance of a bare FTO layer presents only a slight variation as a function of the applied voltage, V app . Similar behaviour is observed for the electrode with a ZrO 2 compact layer (ZZ) and with a nanoporous ZrO 2 layer but no compact layer (0Z). Thus, NS ZrO 2 layers are not charged with the applied bias. Moreover, at high V app , an exponential increase in capacitance is observed for the electrode with only the TiO 2 compact layer (T0), corresponding to the chemical capacitance of the compact TiO 2 (refs 18 , 19 ). The increase in capacitance is higher for the electrode with a NS layer of TiO 2 (TT) as well because of the higher TiO 2 volume compared with the T0 electrode. Contrary to ZrO 2 , TiO 2 can be charged. The chemical capacitance pattern reflects the exponential TiO 2 DOS [18] , [19] . As the V app is increased, charge is accumulated in the TiO 2 DOS but not in ZrO 2 . Only when the TiO 2 compact layer is used with a ZrO 2 nonporous electrode (TZ) can the exponential increase in the chemical capacitance be observed, corresponding to the chemical capacitance of TiO 2 compact layer, as can be inferred from the results in Fig. 2 . This analysis gives an additional proof that no charge is accumulated into ZrO 2 . In this case, ZrO 2 acts as a scaffold for perovskite similar to Al 2 O 3 in previous reports [6] , [9] . 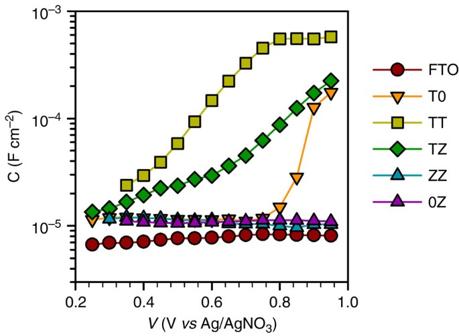Figure 2: Capacitance of non-sensitized electrodes. Capacitance has been extracted from IS measurements in liquid electrolyte with I-/I3-redox couple. Capacitance of the bare conductive SnO2:F (FTO) electrode is compared with electrodes with different layers of TiO2and ZrO2. The electrodes are called using the notation XY, where X is a compact layer, Y is a porous layer and T and Z are TiO2and ZrO2layers, respectively. 0 indicates no layer – that is, T0 compact TiO2layer with no nanoporous layer. Figure 2: Capacitance of non-sensitized electrodes. Capacitance has been extracted from IS measurements in liquid electrolyte with I - /I 3- redox couple. Capacitance of the bare conductive SnO 2 :F (FTO) electrode is compared with electrodes with different layers of TiO 2 and ZrO 2 . The electrodes are called using the notation XY, where X is a compact layer, Y is a porous layer and T and Z are TiO 2 and ZrO 2 layers, respectively. 0 indicates no layer – that is, T0 compact TiO 2 layer with no nanoporous layer. Full size image IS interpretation On the basis of J–V curves alone it is difficult to extract conclusions about the mechanism that determines the different behaviours observed among the different electrodes analysed. Decoupling the effect on the J–V curve of each part of the device merely with this characterization cannot be performed in a straightforward manner, and many times it is impossible. Nevertheless, IS is a frequency characterization technique that allows the decoupling of physical processes with different characteristic times [19] . Its interpretation is not trivial, but once the appropriate models are developed this technique allows separate characterization of each part of the full device at cell working conditions. We have employed this method to analyse the prepared solar cells under dark and one-sun illumination conditions. Here we have focused on the determination of charge accumulation, which is strictly needed for the photovoltaic process. The detailed analysis of all aspects of the impedance spectra is beyond the scope of this communication. Nevertheless, we have developed an advanced model that allows the extraction of all relevant information from the impedance spectra, taking into consideration some previous results on DSSCs [20] . All details on the IS model employed for the characterization of the measured samples can be found in Supplementary Note 1 . Fig. 3 shows an example of the Nyquist plots obtained for the analysed cells. The results correspond to those for NS TiO 2 and ZrO 2 solar cells under both dark and illuminated conditions, both at V app =0 and 0.8 V. The first remarkable fact is that, despite the clear differences between TiO 2 and ZrO 2 electrodes, as discussed previously ( Fig. 2) , similar impedance patterns are obtained for both electrodes. The appearance of a transmission line (TL) under dark and low V app conditions, characterized by a straight line followed by an arc, is also significant (see Fig. 3a,b) . TL is the classical feature seen in NS electrodes, in which transport is coupled with recombination [21] , see Supplementary Fig. S9 . However, this feature is usually not seen for very thin NS TiO 2 electrodes ( Fig. 3 , see Table 1) , and electrodes thicker than 2–3 μm are needed to appreciate this feature. These two facts indicate that new behaviours, in comparison with conventional SSCs, can be attributed to NS perovskite solar cells. 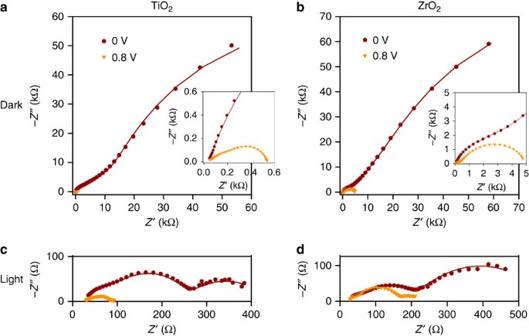Figure 3: Nyquist plots of lead iodine PS solar cells in TiO2and ZrO2electrodes. Nyquist plot of solar cells prepared as FTO/compact TiO2/nanostructured oxide/PS/spiro-MeOTAD/Au. The left column corresponds to the device using TiO2as the NS oxide, whereas the right column corresponds to the device with ZrO2, as shown inFig. 1and summarized inTable 1. (a) and (b) correspond to IS measurements under dark conditions; transmission line behaviour is clearly visible. The inset is a zoom of the low impedance region. (c) and (d) correspond to measurements under 1-sun illumination. Nyquist plots for two different applied DC signals,Vapp, are shown in the graphs. Solid lines are the fits obtained using equivalent circuits previously used for solid DSSC with spiro-MeOTAD,22and in some cases additional R–C feature to the TL for an accurate fitting, seeSupplementary Fig. S9. Figure 3: Nyquist plots of lead iodine PS solar cells in TiO 2 and ZrO 2 electrodes. Nyquist plot of solar cells prepared as FTO/compact TiO 2 /nanostructured oxide/PS/spiro-MeOTAD/Au. The left column corresponds to the device using TiO 2 as the NS oxide, whereas the right column corresponds to the device with ZrO 2 , as shown in Fig. 1 and summarized in Table 1 . ( a ) and ( b ) correspond to IS measurements under dark conditions; transmission line behaviour is clearly visible. The inset is a zoom of the low impedance region. ( c ) and ( d ) correspond to measurements under 1-sun illumination. Nyquist plots for two different applied DC signals, V app , are shown in the graphs. Solid lines are the fits obtained using equivalent circuits previously used for solid DSSC with spiro-MeOTAD, [22] and in some cases additional R–C feature to the TL for an accurate fitting, see Supplementary Fig. S9 . Full size image The capacitance and DOS The direct fingerprint of charge accumulation should be observed in the capacitance, as chemical capacitance reflects the capability of a system to accept or release additional carriers because of a change in its Fermi level [18] . The Nyquist plots in Fig. 3 present a rich impedance pattern with several features. It is not possible to determine in a straightforward manner the part of the IS spectra that contains information about chemical capacitance, see Supplementary Note 1 for further discussions. The IS spectra have been fitted using equivalent circuits previously used for solid DSSC utilizing spiro-MeOTAD [22] . The use of spiro-MeOTAD as the HTM adds an extra degree of complexity to the analysis, as has been pointed out recently [23] , and in some cases it introduces an additional R–C feature to the TL circuit. By focusing on the spectra under illumination conditions, Fig. 3 c, d, we can identify three regions at high, intermediate and low frequencies, hereafter called hf , if and lf , respectively. Considering these features, capacitance of different electrodes has been determined from the if region, see Supplementary Note 1 . From the general information gathered from IS analysis of DSSC, it is well established that the compact layer generally used to cover the conducting glass has a large effect on the capacitance when the interface is polarized at reverse or moderate forward bias. It is therefore important to analyse such layers using Flat samples in order to separately determine the capacitance contribution of the NS layers, which are the active photovoltaic layers. Fig. 4 shows the capacitance extracted from the IS spectra fitting for Flat and NS samples with and without perovskite for both TiO 2 and ZrO 2 electrodes. The left graph includes Flat and blank NS samples (without perovskite) and the right graph includes NS solar cells with perovskite. In the left graph of Fig. 4 , two regions, independent of the NS film material, can be appreciated. One at low V app , V app <0.6–0.7 V, and the other at high V app . For Flat samples at low V app , the growth of capacitance with voltage is moderate and in Fig. 4 it is seen as being practically constant with the logarithmic scale employed in the representation (see red dashed line used as eye guide). At high V app , an increase in the capacitance slope is observed. This exponential enhancement of capacitance can be attributed to the chemical capacitance of the flat TiO 2 compact layer, as it has been pointed out in Fig. 2 for the T0 electrode with only a TiO 2 compact layer. Moreover, the less-voltage-dependent capacitance at low V app could be related to the capacitance of the spiro-MeOTAD with some contribution from the interface capacitance at compact TiO 2 /spiro-MeOTAD [24] . We consider that the role of perovskite in this capacitance is minor (just reducing the compact TiO 2 /spiro-MeOTAD interface effective area), as the amount of perovskite involved is minimal. Confirming this aspect, we observed a similar behaviour for perovskite-free (blank) NS samples independently of the NS layer material TiO 2 or ZrO 2 . For blank NS samples an increase in capacitance at high V app is also observed, and it is more significant for NS TiO 2 , as in this case the chemical capacitance of the NS TiO 2 layer also participates, as has been shown in Fig. 2 . Note that, with the experimental procedure reported in the Methods section for the preparation of CH 3 NH 3 PbI 3 , the amount of perovskite deposited in Flat samples is low and is not enough to produce a distinguishable continuous thin layer of perovskite as can be observed in SEM pictures in Supplementary Fig. S3 . This fact prevented the investigation of the capacitance of thicker CH 3 NH 3 PbI 3 layers. 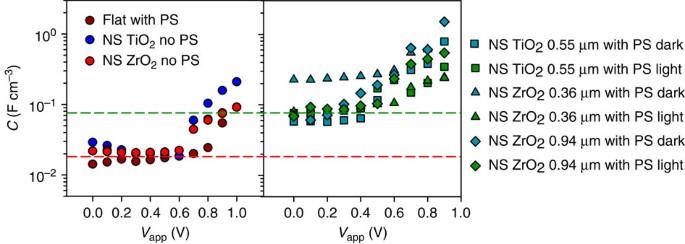Figure 4: Capacitance analysis of flat samples and NS samples with and without PS. The left graph plots capacitance of flat with PS, and blank samples without PS, NS TiO2and ZrO2samples present NS layers of 0.35 μm TiO2and 0.39 μm ZrO2, respectively. The right graph plots the capacitance of NS TiO2and ZrO2samples with PS of samples with different NS layer thicknesses as indicated in the legend. Capacitance values obtained in measurements under dark and under 1-sun illumination (light) conditions are plotted. Capacitance for both graphs has been extracted by fitting the IS spectra from theifregion as discussed inSupplementary Note 1. Capacitance has been normalized to the electrode volume. Red and green dashed lines are only eye guides to highlight the difference in capacitance obtained for samples with and without PS. Figure 4: Capacitance analysis of flat samples and NS samples with and without PS. The left graph plots capacitance of flat with PS, and blank samples without PS, NS TiO 2 and ZrO 2 samples present NS layers of 0.35 μm TiO 2 and 0.39 μm ZrO 2 , respectively. The right graph plots the capacitance of NS TiO 2 and ZrO 2 samples with PS of samples with different NS layer thicknesses as indicated in the legend. Capacitance values obtained in measurements under dark and under 1-sun illumination (light) conditions are plotted. Capacitance for both graphs has been extracted by fitting the IS spectra from the if region as discussed in Supplementary Note 1 . Capacitance has been normalized to the electrode volume. Red and green dashed lines are only eye guides to highlight the difference in capacitance obtained for samples with and without PS. Full size image In the case of complete NS devices with perovskite (right graph Fig. 4) , a clear difference in the capacitance value is observed, obtaining higher capacitances for samples with perovskite than for blank samples (see red and green dashed lines in Fig. 4) . It is worth pointing out that the normalized capacitance is independent of the electrode material (TiO 2 or ZrO 2 ), the NS layer thickness and the illumination conditions at which the IS characterization was carried out (only NS ZrO 2 , 0.35 μm thickness, under dark conditions separates from the general trend at low V app ). This observation indicates that the capacitance observed in this case is neither the interfacial capacitance at the compact TiO 2 interface nor the spiro-MeOTAD nor the TiO 2 (compact or NS) chemical capacitance, or at least not only the TiO 2 chemical capacitance, as similar behaviour is observed in ZrO 2 samples. The remaining possibility is that this capacitance is originated by the perovskite deposited in the NS layer. Charge accumulation in perovskite materials is directly observed. As chemical capacitance maps the DOS, the high perovskite capacitance indicates a high DOS density in this material. This is as far as we know the first observation of charge accumulation in the light-absorbing material for NS solar cells using a combination of absorber, ETM and HTM. This conclusion is also supported by the observation of a large capacitance in Flat samples with a thin film of perovskite, as described below. In order to highlight this new feature observed in NS perovskite solar cells, classical all-solid DSSC with dye N719 and spiro-MeOTAD as the HTM has been prepared and characterized (see Supplementary Figs S10 and S11) . The result of the comparison of the capacitance observed for DSSC and the other samples analyzed (with NS TiO 2 or ZrO 2 ) is shown in Fig. 5 . It is well known that the chemical capacitance extracted from DSSC is the chemical capacitance of the NS TiO 2 layer [18] , [19] , [22] . Chemical capacitance of DSSC, obtained from the if region, represented with inverted triangles with a red edge in Fig. 5 , reflects the exponential DOS of TiO 2 . Note the significant difference between the chemical capacitance of DSSC and NS TiO 2 perovskite solar cells (consider only the capacitance extracted at the if region). Only at high V app do both capacitances merge to indicate a possible contribution of both materials, perovskite and NS TiO 2 , to the charge accumulation. In the case of NS ZrO 2 samples with perovskite, the main contribution to the capacitance is from perovskite, but a contribution of compact TiO 2 cannot be ruled out at high V app . These results indicate that, although SSCs and perovskite NS solar cells present similar configuration (when a NS TiO 2 electrode is used), the working principles are different, with charge accumulation and transport in perovskite material exhibiting a very large DOS. Deep knowledge of these working principles of perovskite NS solar cells is mandatory for a further improvement of this new kind of devices. 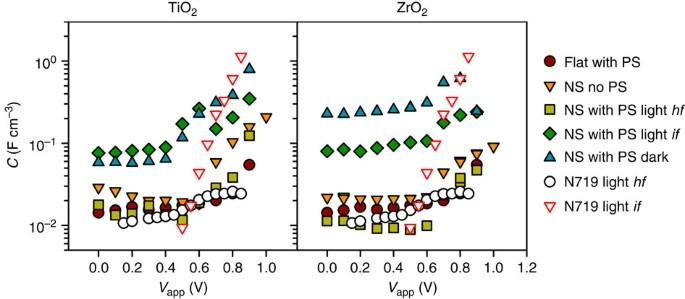Figure 5: Capacitance analysis of TiO2and ZrO2and comparison with a solid DSSC using N719 dye. The left graph plots capacitance of the following: flat sample with PS; blank NS TiO2(0.35 μm thickness) with no PS; NS TiO2(0.55 μm thickness) with PS extracted from measurement under dark and under 1-sun illumination (light) conditions; and all-solid DSSC (2.2 μm thickness) with N719 as dye and spiro-MeOTAD as HTM. The right graph plots capacitance of the following: flat samples with PS; blank NS ZrO2(0.39 μm thickness) with no PS; NS TiO2(0.36 μm thickness) with PS extracted from measurements under dark and under 1-sun illumination (light) conditions; and all-solid DSSC (2.2 μm thickness) with N719 as dye and spiro-MeOTAD as the HTM. Capacitance has been normalized to the electrode volume. Capacitance for both graphs has been extracted by fitting the IS spectra from theifregion if nothing else is indicated. In some cases, capacitance has been extracted from thehfregion as it is indicated in the legend. Figure 5: Capacitance analysis of TiO 2 and ZrO 2 and comparison with a solid DSSC using N719 dye. The left graph plots capacitance of the following: flat sample with PS; blank NS TiO 2 (0.35 μm thickness) with no PS; NS TiO 2 (0.55 μm thickness) with PS extracted from measurement under dark and under 1-sun illumination (light) conditions; and all-solid DSSC (2.2 μm thickness) with N719 as dye and spiro-MeOTAD as HTM. The right graph plots capacitance of the following: flat samples with PS; blank NS ZrO 2 (0.39 μm thickness) with no PS; NS TiO 2 (0.36 μm thickness) with PS extracted from measurements under dark and under 1-sun illumination (light) conditions; and all-solid DSSC (2.2 μm thickness) with N719 as dye and spiro-MeOTAD as the HTM. Capacitance has been normalized to the electrode volume. Capacitance for both graphs has been extracted by fitting the IS spectra from the if region if nothing else is indicated. In some cases, capacitance has been extracted from the hf region as it is indicated in the legend. Full size image Thin-film solar cell As the results reported so far in the literature indicate that the organometal halide perovskite may work both as light absorber and as ambipolar electron and hole transport material, it is of great interest to explore the operation of these materials in thin-film solar cell configurations in which a compact layer is sandwiched between selective contacts. It is important, therefore, to confirm that the distinctive large DOS observed in NS samples is found in planar samples as well. We have commented above on very thin layers of CH 3 NH 3 PbI 3 , but the capacitance results were not conclusive. Therefore, we have also prepared a Flat cell of CH 3 NH 3 PbI 3−x Cl x following a processing method recently reported [8] , obtaining a Flat sample with a perovskite layer of 300 nm. The measurements of capacitance of such thin-film configurations, described in Supplementary Note 2 , indicate a large capacitance that doubtless corresponds to the perovskite layer, see Supplementary Fig. S13 , confirming our results above on the huge intrinsic DOS of this type of materials for NS perovskite samples. In this article we showed for the first time the charge accumulation in light-absorbing materials, CH 3 NH 3 PbI 3 perovskite, in a NS solar cell. High DOS has been observed for perovskite. This direct evidence has been observed by the capacitance extracted from IS measurements for both NS TiO 2 and ZrO 2 electrodes, despite the large differences from the electrical point of view between these two materials. This study indicates that the analysed solar cell constitutes a new kind of photovoltaic device halfway between sensitized and thin-film solar cell for NS TiO 2 and a thin-film solar cell with ZrO 2 scaffold for NS ZrO 2 . The optimization and further improvement of a new photovoltaic technology requires a deep knowledge of the working principles of this photovoltaic device. Understanding how charge accumulation is reached and how it can be identified and characterized is an important step forward, with significant implications on the development of this technology. Electrode preparation and characterization The electrodes analysed in this study include flat and nanoporous morphologies for TiO 2 and ZrO 2 . The semiconductor compact layers (CLs) were prepared by spin-coating a solution of M (IV) bis(ethyl acetoacetato)-diisopropoxide (M=Ti or Zr), 0.15 M, in 1-butanol on fluorine-doped tin oxide (FTO)-covered glass substrates (Pilkington) TEC 15. The coated films were cooled down, and the spin–cast was repeated twice with a double-concentrated precursor solution followed by thermal treatment at 450 °C. The thicknesses determined by scanning electron microscopy were ~100 nm and ~60 nm for TiO 2 and ZrO 2 , respectively. Porous TiO 2 films were prepared using the doctor-blade method with a 20-nm-sized paste prepared according to the method described elsewhere [25] and sintering at 450 °C for 30 min in air. Porous ZrO 2 films were also prepared by means of the doctor-blade method using ZrO 2 paste with a particle size of 15 nm [25] and sintered under the same conditions than porous TiO 2 film. The thicknesses of nanoporous films were ~0.3–2 μm for solar cell characterization and 2–4 μm for electrode characterization. CH 3 NH 3 PbI 3 perovskite precursor solution was prepared by mixing PbI 2 (1.23 mmol, 99%, Aldrich) and CH 3 NH 3 I (1.23 mmol, synthesized) in γ-butyrolactone (1 ml, 99%, Fluka), producing 40 wt% solution. The CH 3 NH 3 I was readily synthesized by reacting CH 3 NH 2 (0.273 mol, 40% in methanol, TCI) with HI (0.227 mol, 57 wt.% in water, Aldrich) according to the method reported elsewhere [5] , [10] . The perovskite precursor solution, kept at 60 °C with stirring for 12 h, was deposited on the prepared flat or nanoporous TiO 2 and ZrO 2 films by spin-coating, which was followed by heating at 100 o C for 15 min. The perovskite-adsorbed films were covered with hole transport material (HTM) using spin-coating, where HTM solution is composed of 0.14 M 2,2′,7,7′-tetrakis-(N,N-di- p -methoxyphenyl-amine)-9,9′-spirobifluorene (spiro-MeOTAD, Merck), 64 mM bis(trifluoromethane)sulfonimide lithium salt (Li-TFSI, 99.95%, Aldrich) and 0.198 M 4- tert -butylpyridine ( t BP, 96%, Aldrich) in a mixture of chlorobenzene (99.8%, Aldrich) and acetonitrile (99.8%, Aldrich) with a volume ratio of 10:1. A 70-nm-thick Au (99.99%) layer as a counter electrode was evaporated on top of the HTM overlayer under ~10 −6 mbar. J–V characteristics of solar cells were determined under 1-sun illumination (AM 1.5 G, 100 mWcm −2 ) with an ABET Sun 2000 solar simulator (1,000W Xe source) and a Keithley 2,400 sourcemeter. Measurements were recorded without a mask. This procedure overestimates the efficiency by ~10% [26] . Photoelectrochemical measurements were recorded using an FRA-equipped PGSTAT-30 from Autolab. A three-electrode configuration was used where a Pt wire was connected as the counter-electrode and Ag/Ag + non-aqueous was used as the reference electrode. Anhydrous and degassed acetonitrile with redox iodide/triiodide (0.5 M LiI, 0.05 M I 2 ) was used as the electrolyte. Cyclic voltammetries were recorded at a scan rate of 50 mV/s and impedance characterization was performed at forward bias, applying a 20 mV AC sinusoidal signal over the constant applied bias with the frequency ranging between 400 kHz and 0.1 Hz. How to cite this article: Kim, H.-S. et al. Mechanism of carrier accumulation in perovskite thin-absorber solar cells. Nat. Commun. 4:2242 doi: 10.1038/ncomms3242 (2013).